Strong interactive growth behaviours in solution-phase synthesis of three-dimensional metal oxide nanostructures Wet-chemical synthesis is a promising alternative to the conventional vapour-phase method owing to its advantages in commercial-scale production at low cost. Studies on nanocrystallization in solution have suggested that growth rate is commonly affected by the size and density of surrounding crystals. However, systematic investigation on the mutual interaction among neighbouring crystals is still lacking. Here we report on strong interactive growth behaviours observed during anisotropic growth of zinc oxide hexagonal nanorods arrays. In particular, we found multiple growth regimes demonstrating that the diameter of the rod is dependent on its height. Local interactions among the growing rods result in cases where height is irrelevant to the diameter, increased with increasing diameter or inversely proportional to the diameter. These phenomena originate from material diffusion and the size-dependent Gibbs–Thomson effect that are universally applicable to a variety of material systems, thereby providing bottom-up strategies for diverse three-dimensional nanofabrication. Precisely controlled growth of one-dimensional nanocrystals (that is, wires, tubes and rods) has created opportunities to fabricate new types of devices with generic vertical configurations possessing advantageous electrical, optical, biological and mechanical properties, as well as high-density integration [1] , [2] , [3] , [4] , [5] . This growth is usually achieved by a vapour-phase deposition method, in which key parameters determining the growth behaviours have been thoroughly investigated. In particular, there has been substantial interest in axial growth rate in correlation with the diameter and interspacing of nanocrystals [6] , [7] , [8] , [9] , [10] , yet experimental results on this topic have varied from case to case, and its mechanism has not been satisfactorily determined thus far. For example, it has been generally accepted that the Gibbs–Thomson (GT) effect leads to a shorter length for smaller diameters [6] , [7] , [8] , but the opposite dependence has also been reported and was ascribed to the role of material diffusion that prevails over interfacial reaction [9] , [10] , [11] , [12] . In particular, when growth occurs via a vapour–liquid–solid process, the crystallization reaction is further mediated by a nanosized catalyst, and the resulting interplay between the incorporation of reactants and crystallization makes the situation more complicated [13] , [14] . Accordingly, despite the fact that growth kinetics provide an additional degree of freedom for three-dimensional (3D) nanofabrication, the overall complexity makes precise control of crystal nanostructures difficult in practice. Moreover, these approaches were generally performed with high-temperature vacuum processing within a narrow growth window, and thus there are critical limits in cost-effective production and controllability. There has been similar interest in solution-phase synthesis due to its simplicity and the capability to produce single-crystalline nanocrystals with controlled orientation, size and morphology [15] , [16] , [17] , [18] , [19] , [20] , [21] . Solution-phase synthesis is also available for epitaxial growth if the conditions are set to allow for heterogeneous solidification to take place at a low level of supersaturation [22] , [23] , [24] . This approach is further exemplified herein to achieve patterned arrays of vertically grown ZnO hexagonal rods. In the synthesis, strong interactions among the adjacent crystals, originating from GT, competitive and/or synergetic effects, are found to produce diverse relationships between diameter and axial growth velocity. Systematic study is performed to understand multiple types of growth mechanisms, and significant dependence of the rod diameter on the height. These unique behaviours are further exploited to construct more sophisticated nanostructures with artificially regulated 3D height profiles. Growth behaviours with different solute concentration Solution-phase synthesis of ZnO rods is based on a hydrothermal reaction process involving the dissociation of zinc nitrate and hexamethylenetetramine (HMT) that produces Zn 2+ and hydroxyl (OH − ) ions, respectively [25] . As a polar crystal comprised of tetrahedrally coordinated Zn 2+ and O 2− ions, the preferential growth along the c axis orientation continues by iterative reaction involving association and dehydration of the precursor ions at the top (0001) surfaces. The precipitation occurs either directly (that is, Zn 2+ +2OH − ↔Zn(OH) 2 ↔ZnO s +H 2 O) or via the zinc hydroxide (that is, Zn 2+ +2OH − ↔Zn(OH) 2 ↔ZnO s +H 2 O), depending on the solution conditions [26] . Heating of the solution is required to activate the chain of processes, but growth usually occurs below the boiling point of water. Due to the low growth temperature as well as site-specific capture of ions, size- and position-controlled growth could be achieved by lithographically defined polymer patterns on a ZnO seed layer ( Fig. 1d ) [27] . We first grew ZnO rods via polymethylmethacrylate (PMMA) patterns consisting of circular hole arrays, in which the diameter in columns increased from 100 to 600 nm while the centre-to-centre distance L c–c was set to 800 nm (see Methods for details). The resulting ZnO rods have near-perfect vertical alignment and in-plane hexagonal symmetry, as confirmed in the scanning electron microscopy images in Fig. 1a–c . In addition, although diameter D ZnO (that is, hexagon diagonal) and height H ZnO are sensitive to the growth parameters, they are relatively uniform for growth from holes of the same size under identical conditions with average s.d. of ~4% in diameter and ~2% in height. 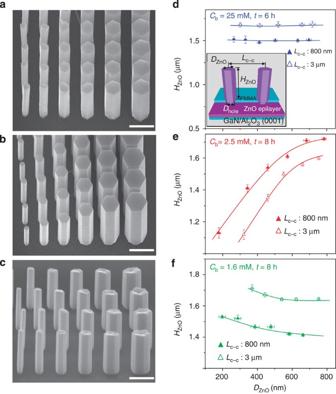Figure 1: Height versus diameter for ZnO rod arrays grown with different solute concentrations. (a–c) Scanning electron microscopy (SEM) images of ZnO hexagonal rod arrays with different solute concentrations,Cb, revealing the existence of three different growth regimes characterized by the interplay between the diameterDZnOand heightHZnO: (a) at aCbof 25 mM,HZnOis irrelevant toDZnO; (b) at aCbof 2.5 mM,HZnOincreases with increasingDZnO; (c) at aCbof 1.6 mM,HZnOdecreases with increasingDZnO. The images were taken at the tilt angles of 30° (aandb) and 70° (c). For patterned growth, circular hole arrays with the diameters in columns increased from 100 to 600 nm for a constant centre-to-centre distanceLc–cof 800 nm were used as masks (seeSupplementary Fig. 1, type I). Scale bars, 1 μm. The growth times (t) were 6 h for the sample inaand 8 h for the samples inbandc. (d–f) Plots ofHZnOversusDZnOfor the ZnO rods grown atCbvalues of 25 mM (d), 2.5 mM (e) and 1.6 mM (f). The holes in the growth masks are identical to those used inbandc, except forLc–c. In the plots, closed triangles with solid trend lines correspond to an LC–Cof 800 nm, and open triangles with solid trend lines correspond to anLc–cof 3 μm. Inset indis the schematic illustrating geometry and definitions of the parameters used in this study. All error bars denote 1 s.d. from the average of more than 10 rod measurements. Figure 1: Height versus diameter for ZnO rod arrays grown with different solute concentrations. ( a – c ) Scanning electron microscopy (SEM) images of ZnO hexagonal rod arrays with different solute concentrations, C b , revealing the existence of three different growth regimes characterized by the interplay between the diameter D ZnO and height H ZnO : ( a ) at a C b of 25 mM, H ZnO is irrelevant to D ZnO ; ( b ) at a C b of 2.5 mM, H ZnO increases with increasing D ZnO ; ( c ) at a C b of 1.6 mM, H ZnO decreases with increasing D ZnO . The images were taken at the tilt angles of 30° ( a and b ) and 70° ( c ). For patterned growth, circular hole arrays with the diameters in columns increased from 100 to 600 nm for a constant centre-to-centre distance L c–c of 800 nm were used as masks (see Supplementary Fig. 1 , type I). Scale bars, 1 μm. The growth times ( t ) were 6 h for the sample in a and 8 h for the samples in b and c . ( d – f ) Plots of H ZnO versus D ZnO for the ZnO rods grown at C b values of 25 mM ( d ), 2.5 mM ( e ) and 1.6 mM ( f ). The holes in the growth masks are identical to those used in b and c , except for L c–c . In the plots, closed triangles with solid trend lines correspond to an L C–C of 800 nm, and open triangles with solid trend lines correspond to an L c–c of 3 μm. Inset in d is the schematic illustrating geometry and definitions of the parameters used in this study. All error bars denote 1 s.d. from the average of more than 10 rod measurements. Full size image Interestingly, the growth of ZnO rods is sensitive to solute concentration C b , as characterized by the correlation between D ZnO and H ZnO . ZnO rod arrays grown at a C b above 25 mM show that the H ZnO is nearly independent of D ZnO ( Fig. 1a ), while H ZnO increases with increasing D ZnO for the sample grown at an intermediate C b of 2.5 mM ( Fig. 1b ); if the C b decreases further to 1.6 mM, thinner rods become longer than thicker rods ( Fig. 1c ). Growth under surface reaction-limited conditions Solution-phase synthesis is analogous to vapour-phase growth, in that the reaction at the solid surface or mass transport through the boundary layer is rate limiting. Given that higher C b provides a sufficient supply of precursor ions, the growth at higher C b ( C b =25 mM) becomes more surface reaction dependent. In this growth regime, growth of rods is hardly affected by neighbouring rods. Notably, the GT effect, wherein the driving force for the phase transformation (that is, axial growth) is size dependent, is negligible ( Fig. 1a,d ). GT effect under mass transport-limited conditions On the other hand, growth rate of ZnO rods becomes dependent on D ZnO with reduced C b . When the precursor concentration decreased by a factor of 10 ( C b =2.5 mM), growth showed such a strong diameter dependence that the rods with an 800-nm diameter are roughly twice as high as those with a 200-nm diameter ( Fig. 1b,e ). The reduced supply of precursors makes growth more sensitive to mass transfer of the precursor ions. Under these circumstances, individual rods do not behave anymore as independent objects and interfere with each other, especially where the inter-rod spacing is much smaller than the thickness of the boundary layer formed over the substrate surface. We attribute this phenomenon mainly to the differences in local equilibrium concentration of the precursors in the regions of rods with different sizes. This is based on the GT effect, which generates increases in local concentration relative to the equilibrium concentration at a flat surface [28] (radius of curvature r =∞) that are inversely proportional to the radius of crystal curvature, r ZnO . The resulting concentration gradients cause a flux of precursor ions from the regions of thin rods to regions of thicker ones, thereby leading to diameter dependence of the growth velocity. An extreme case of the GT effect is Ostwald ripening [29] , [30] , [31] , in which the capillary forces cause larger-sized crystals to grow at the expense of smaller-sized crystals. Source competition under mass transport-limited conditions If C b is further decreased below 1.6 mM, the situation is reversed in that H ZnO is inversely proportional to D ZnO ( Fig. 1c,f ). This phenomenon originated from an increased competition for the precursor among the neighbouring rods [9] , [10] . Thicker rods need more precursor consumption to grow at the same rate as thinner rods, but the limited precursor ions available from the surroundings lead to a decrease in growth rates. The competition is still active at a lower solute concentration of 1.25 mM or at a wider rod-to-rod spacing L c–c of 3 μm ( Fig. 1f ). Another distinct feature is that the thick rods grown in this situation generally have a concave tip, which should be related to the transport of Zn 2+ ions and/or their local distributions due to the electrostatic interaction near the top polar surface of ZnO rods that are more critical in the competition regime. There should be a localized increase in the Zn 2+ ion concentration at the edge of the surface compared with the centre, since the surface polarity is stronger at the centre of tips [32] . In addition, Zn 2+ ions existing in the surrounding diffuse along the nonpolar side surface or in the solution and mostly arrive at the edge of the tips earlier than at the centre [25] , [27] . As a consequence, precipitation occurs preferentially at the edge of the tips, which produces their unique morphology. A similar mechanism was introduced to explain the ZnO nanotube growth in solution [32] . In our model, mutual interactions among growing rods might not only be determined by D ZnO and synthesis parameters, but can also be affected by inter-distances and configurations of the neighbouring crystals. To clarify this issue and to investigate the change in growth velocities of ZnO rods depending on the configurations, we grew a series of square arrays (6 × 10) of ZnO rods using circular hole arrays with diameters that gradually increased from 100 nm (far left array) to 500 nm (far right array) ( Fig. 2a,b ) while being identical within the same array. At C b of 2.5 mM (in which the GT effect dominates), the H ZnO shows a gradual increase with D ZnO , but it becomes saturated when thicker rods are closely adjacent and the gaps between the rods are smaller than D ZnO ( D ZnO ≥500 nm) ( Fig. 2c , red squares). This can be attributed to the onset of material competition, counteracting the local concentration gradient originating from the GT effect. Along the same lines, for the case of C b below 1.6 mM (in the competition control regime), the more severe competition among the thicker rods caused a further decrease in the growth rate. Consequently, H ZnO became more sensitive to D ZnO for the square arrays (green and blue squares in Fig. 2c ), compared with those in Fig. 1f (see also Supplementary Fig. 8 ). 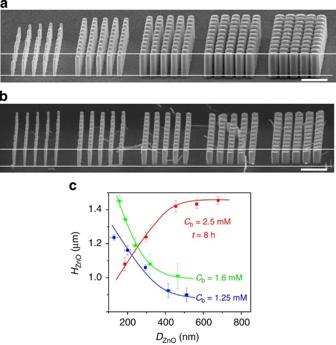Figure 2: Gibbs–Thomson and competition effects in square arrays of ZnO rods. (a–b) Scanning electron microscopy images (70° tilt view) of square arrays (6 × 10) of ZnO rods grown at aCbof 2.5 mM (a) and 1.6 mM (b). For the growth mask, circular hole arrays with diameters (identical in the same arrays) gradually increasing from 100 nm (far left array) to 500 nm (far right array) were used (seeSupplementary Fig. 1, type II). Scale bars, 2 μm. (c) Plots ofHZnOversusDZnOfor the series of square arrays (6 × 10) of ZnO rods. Holes in the growth masks are identical to those used inaandb. All error bars denote 1 s.d. from the average of more than 10 rod measurements. Figure 2: Gibbs–Thomson and competition effects in square arrays of ZnO rods. ( a – b ) Scanning electron microscopy images (70° tilt view) of square arrays (6 × 10) of ZnO rods grown at a C b of 2.5 mM ( a ) and 1.6 mM ( b ). For the growth mask, circular hole arrays with diameters (identical in the same arrays) gradually increasing from 100 nm (far left array) to 500 nm (far right array) were used (see Supplementary Fig. 1 , type II). Scale bars, 2 μm. ( c ) Plots of H ZnO versus D ZnO for the series of square arrays (6 × 10) of ZnO rods. Holes in the growth masks are identical to those used in a and b . All error bars denote 1 s.d. from the average of more than 10 rod measurements. Full size image Synergetic effect In the GT control regime (at C b of 2.5 mM), the overall H ZnO values decreased by ~0.2 μm with increasing L c–c from 800 nm to 3 μm (see closed versus open triangles in Fig. 1e ; Fig. 3a,b also directly compares the heights of rods with the same D ZnO , but different values of L c–c ). This is contrary to the cases at lower C b , where the contribution of source sharing results in higher growth rate at wider rod-to-rod spacings ( Fig. 1f , see also Supplementary Figs 2 and 3 ). Similar behaviour was observed during vapour-phase growth of III–V compound nanowires and was attributed to the catalysed decomposition of metal-organic precursors to secondary species that diffused to neighbouring wires and synergistically contribute to wire growth [33] . As mentioned earlier, in our case, ZnO can be precipitated via the hydroxide, which illustrates the development of the Zn(OH) 2 at the rod surfaces, especially at the tips. The intermediate specie is known to be stable in an aqueous solution at a relatively high ion concentration [32] , [34] , and can be desorbed or reabsorbed reversibly and contribute to the growth of neighbouring rods within their diffusion limit. The Zn(OH) 2 , however, dissolves easily in lower ion concentration, and thereby the synergetic effect is not significant in the competition regime. 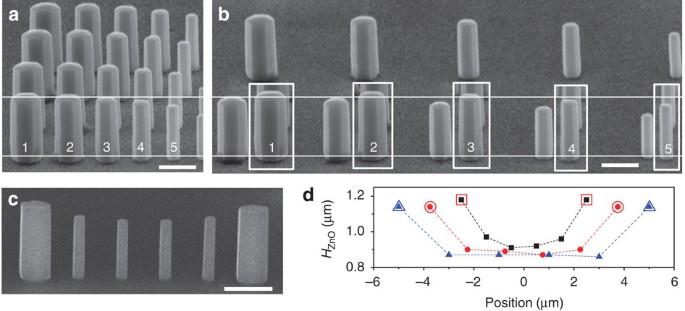Figure 3: Analysis of the synergetic effect. (a–b) Scanning electron microscopy (SEM) images (70° tilt view) of ZnO rod arrays with diameters in column gradually decreasing from 800 to 200 nm atLc–cof 800 nm (a) andLc–cof 3 μm (b).Cbis set to 2.5 mM for both cases. For direct comparison, each image of rods inais inserted right after the corresponding rods with the same diameters (white boxes inb). Scale bars, 1 μm. (c) SEM image of linear arrays of small diameter rods (DZnO=230 nm) between thicker rods (DZnO=625 nm) with anLc–cof 1 μm (seeSupplementary Fig. 1, type III). Scale bar, 1 μm. (d) Plot ofHZnOas a function of position with differentLc–cvalues (black square: 1 μm; red circle: 1.5 μm; blue triangle: 2 μm). ForLc–c≤1.5 μm, thin rods (DZnO=230 nm) immediately adjacent to thicker rods (DZnO=625 nm, marked with larger open symbols) are taller than those in the middle of the array. Figure 3: Analysis of the synergetic effect. ( a – b ) Scanning electron microscopy (SEM) images (70° tilt view) of ZnO rod arrays with diameters in column gradually decreasing from 800 to 200 nm at L c–c of 800 nm ( a ) and L c–c of 3 μm ( b ). C b is set to 2.5 mM for both cases. For direct comparison, each image of rods in a is inserted right after the corresponding rods with the same diameters (white boxes in b ). Scale bars, 1 μm. ( c ) SEM image of linear arrays of small diameter rods ( D ZnO =230 nm) between thicker rods ( D ZnO =625 nm) with an L c–c of 1 μm (see Supplementary Fig. 1 , type III). Scale bar, 1 μm. ( d ) Plot of H ZnO as a function of position with different L c–c values (black square: 1 μm; red circle: 1.5 μm; blue triangle: 2 μm). For L c–c ≤1.5 μm, thin rods ( D ZnO =230 nm) immediately adjacent to thicker rods ( D ZnO =625 nm, marked with larger open symbols) are taller than those in the middle of the array. Full size image On the basis of our hypothesis, the synergetic effect becomes significant when rods are located close enough without substantial overlap of the precursor collection volumes, and thus precursor competition is negligible. To examine the validity of the hypothesis, we grew linear arrays of small diameter rods ( D ZnO =230 nm) between thicker rods ( D ZnO =625 nm). When the rods are located at an L c–c of 1 μm, thin rods right next to the thick rods grew faster than those in the middle of the array ( Fig. 3c ); this is a characteristic feature of the synergetic effect of crystal growth [33] , [35] . It is also noted that both thicker rods and neighbouring thinner rods accelerate each others’ growth rate, resulting in an overall increase in the H ZnO ( Fig. 3d ). As expected, the synergetic effect decreases with increasing inter-rod spacing and, in this case, almost disappeared at an L c–c of 2 μm or longer, whereas the GT effect is still strongly active. We attribute our finding on strong interactive growth to complex interplay of diffusing transport of precursor ions and Zn(OH) 2 around the neighbouring rods. To justify our growth model, the contribution of local diffusion of Zn 2+ ions between the neighbouring rods, J i , relative to bulk diffusion through the boundary layer, J b , is first considered numerically. Under quasi-steady-state conditions, the precursor ion concentration in the boundary layer decreases linearly and comes close to C si = C bi /(1+Φ) near the flat solid surface, where C bi is the ion concentration in the bulk solution and the Thiele modulus (Φ) is the ratio of the surface reaction rate to the diffusion rate. If the size effect was taken into account, the local equilibrium concentration near the surface of the rod with a radius of curvature r ZnO slightly increases to by the GT effect, where γ is the interfacial energy, V m is the molar volume of the solid phase, R is the gas constant and T is the temperature [28] . In the case of Ф<1 (at higher C bi ), the overall growth is determined by consumption rate via surface reaction, J s , and thus the local concentration difference between the rod surfaces has no substantial influence. However, in the mass transport-limited regime (Ф>1), the interplay between bulk and local diffusion prevails over surface reaction, and their contributions are simply estimated as a function of Ф (see Supplementary Methods and Supplementary Fig. 10 for details). The ratio of J i to J b for the adjacent rods with D ZnO of 800 and 140 nm, respectively, separated by 1–3 μm, is shown in Fig. 4 , in which lateral growth is ignored. The boundary layer thickness δ was set to a typical diffusion length of Zn 2+ ions (~300 μm). Importantly, the J i / J b becomes larger for smaller Ф and, as Ф approaches 1, J i / J b reaches 1.6 even at a wider L c–c of 3 μm. We therefore conclude that the GT effect has a crucial influence to yield the strong diameter-dependent height profile observed in this study. Conversely, with reduced C bi (Ф>>1), J i becomes negligible compared with J b , while competition for the precursor consumption increases. Accordingly, this leads to a complete reversal of the D ZnO – H ZnO relationship, as observed for C b below 1.6 mM. 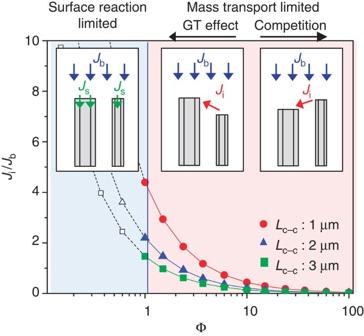Figure 4: Interplay between bulk diffusion and local diffusion. The ratio ofJbandJias a function of Thiele modulus, Ф, under quasi-steady-state conditions. In the surface reaction-limited regime (Ф<1), rod growth is governed by surface reaction rateJs. In the mass transport-limited regime (Ф>1), the contribution ofJibecomes important for smaller values of Ф, but becomes negligible for Ф>>1, while completion for precursor consumption increased with increasing Ф. In this calculation, the synergetic effect was not considered. Figure 4: Interplay between bulk diffusion and local diffusion. The ratio of J b and J i as a function of Thiele modulus, Ф, under quasi-steady-state conditions. In the surface reaction-limited regime (Ф<1), rod growth is governed by surface reaction rate J s . In the mass transport-limited regime (Ф>1), the contribution of J i becomes important for smaller values of Ф, but becomes negligible for Ф>>1, while completion for precursor consumption increased with increasing Ф. In this calculation, the synergetic effect was not considered. Full size image On the other hand, given that the J i / J b is inversely proportional to the L c–c , a stronger GT effect is expected by reducing the L c–c . This is, however, somewhat mismatched with our observation. For example, the height difference between different diameter rods is almost unaffected by L c–c (in case of Fig. 1e ) or slightly reduced at lower L c–c (in case of Fig. 3d ). To explain this, diffusive transport of the Zn(OH) 2 also must be considered. According to the aforementioned synergetic effect, intermediate species are generated near the top (0001) surfaces of thicker rods and enhance the axial growth of nearby thinner rods, compensating for the height difference driven by the GT effect. It should be noted that the concentration of the intermediate species is higher at the rod surface than in the surroundings; thereby, they diffuse circumferentially (that is, the flux is inversely proportional to L c–c n ; n ~3). This is different from the case of Zn 2+ ions, whose concentration is lower at the rod surface (which acts as a sink) than the surroundings (see Supplementary Fig. 4 ); here, diffusion of Zn 2+ ions caused by the GT effect occurs mainly between adjacent rods with different diameters (that is, J i is inversely proportional to L c–c n ; n ~1) under equilibrium conditions. This analysis also explains the rapid disappearance of the synergetic contribution, with an effective range of the Zn(OH) 2 of <~2–3 μm; this is significantly lower than that of precursor Zn 2+ ions. Although our simple analyses partly illustrate the complicated interaction among the growing crystals, further theoretical studies are needed to improve our fundamental understanding on these phenomena and to provide a generic model that will be applicable to various material systems. Investigations on the ZnO crystal growth in solution have shown that the concentrations of reactant species would evolve with a prolonged growth time [26] , [36] , which could affect the growth kinetics. To address this issue, we have investigated the time dependence of H ZnO on D ZnO at various precursor concentrations (see Supplementary Figs 5–7 ). In all cases ( C b =25, 2.5 and 1.6 mM), the growth rate is relatively slow at the initial stage ( t <1–2 h). This is attributed to the diffusion barrier created by the PMMA holes and/or nucleation barrier that exists even in homoepitaxial growth [37] . Following the initial stage, the growth rate becomes faster and stabilized. At C b of 25 mM, H ZnO is almost irrelevant to D ZnO during the entire growth process (over up to 10 h) ( Supplementary Fig. 5a ). At C b of 2.5 mM, there is no dependence of H ZnO on D ZnO in the beginning ( t <2 h), but thereafter the H ZnO significantly depends on D ZnO because the GT effect becomes dominant ( Supplementary Fig. 5b ). More interestingly, at C b of 1.6 mM, H ZnO increases with increasing D ZnO in the beginning ( t <~6 h), but afterwards the situation is gradually reversed ( Supplementary Figs 5c and 7 ); such a gradual change of the growth behaviour from the GT to the competition regimes is associated with the decreasing precursor concentration with time [26] . To further demonstrate the general applicability of our findings, we tested the growth of ZnO nanostructures with more complicated patterns, targeting specific 3D geometries. Growth in GT effect-dominating conditions allows thick rods to grow longer and produces castle-like 3D nanostructures. It is also possible to produce an inverted high profile in the competition regime ( Fig. 5 ). Such 3D nanoarchitectures provide unique applications that would be difficult to be achieved by top-down fabrication approaches or that may require multiple-stage repetitive processing. As a proof of concept for practical applications, Si nanotube arrays were fabricated by employing a ZnO rod array as a sacrificial template, and they then served as an active constituent of highly sensitive strain gauges (or pressure sensors) (see Methods and Supplementary Fig. 9 ). This new type of electronic sensor can enable stepwise response to nanoscale deflection owing to the nanoscale height profile of the 3D Si nanotube array. 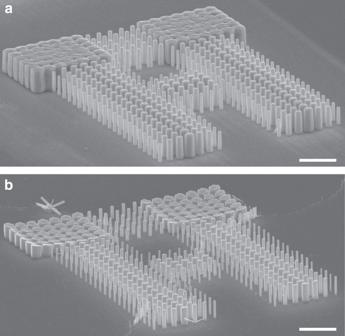Figure 5: Solution-phase fabrication of 3D ZnO nanoarchitectures. (a) Castle-like 3D ZnO nanostructures grown in the GT-effect regime. (b) ZnO nanostructures grown with an identical mask but in the competition regime resulted in an inverted high profile. Scale bars, 3 μm. Figure 5: Solution-phase fabrication of 3D ZnO nanoarchitectures. ( a ) Castle-like 3D ZnO nanostructures grown in the GT-effect regime. ( b ) ZnO nanostructures grown with an identical mask but in the competition regime resulted in an inverted high profile. Scale bars, 3 μm. Full size image In summary, we demonstrated multiple types of growth mechanisms showing significant dependence of the diameter of the ZnO rod on the height, and elucidated the strong interactive growth behaviours observed in the anisotropic growth of these nanocrystal arrays. In this stage, our study is restricted to the case of ZnO crystals; however, this has its origin in general phenomena, including diffusion and the GT effect, which can be commonly applicable to a variety of materials, and thereby represents an opportunity for ab initio synthesis of diverse and functional 3D nanostructures in the solution phase. Hydrothermal growth of ZnO rod arrays For epitaxial growth of ZnO hexagonal rods, ZnO epilayers grown on GaN films on Al 2 O 3 (0001) substrates were used as a seed layer. First, native oxide on a GaN surface was removed via chemical etching with aqua regia containing (3 HCl: 1 HNO 3 ) for 5 min. Then, ZnO seed layers were deposited at 450 °C by metal-organic chemical vapour deposition (MOCVD), which produced c axis-oriented ZnO films with a typical thickness of ~200 nm. A detailed experimental description of the MOCVD process of ZnO films can be accessed elsewhere [27] . To achieve position and diameter-controlled growth of ZnO rod arrays, ~120-nm-thick PMMA mask layers were spin-coated on the ZnO seed layers, and then arrays of circular holes were defined using an electron beam lithography technique. The geometries and parameters of hole arrays used in this study are schematically shown in Supplementary Fig. 1 . For the solution-phase synthesis of ZnO rods, aqueous solutions containing equimolar concentrations of zinc nitrate hexahydrate (ZNH) (Zn(NO 3 ) 2 .6H 2 O, Sigma-Aldrich) and HMT (C 6 H 12 N 4 , Sigma-Aldrich) were used. The mixture solution of 25 mM ZNH and 25 mM HMT was diluted by adding appropriate volumes of deionized water to control the solute concentration in the range of 25–1.6 mM. Finally, the samples of ZnO seed layers coated with PMMA patterns were immersed into the prepared aqueous solutions, and they were then placed in an oven at 70 °C. Fabrication of nano-strain gauge devices Nano-strain gauge devices were fabricated using the following procedures: first, patterned ZnO rod arrays with different D ZnO (from 200 to 600 nm) and H ZnO (from 480 to 510 nm) were coated with a thin Si layer (typically 50 nm thick) by CVD. The thin Si layer, that is, a Si membrane with a 3D nanotube array at its centre, was then coated with a thin protecting layer of PMMA. By submerging the sample in HF solution (50 wt% diluted 1:20 v/v in deionized water), the core ZnO template was selectively etched, which separated the PMMA/Si membrane from the substrate. After rinsing with deionized water, the freestanding PMMA/Si membrane was mounted on the device substrate (plastic or Si/SiO 2 substrate), in which the metal bottom electrode was pre-defined. Using an electron beam lithography technique, a trench was defined at the central region of PMMA where the Si nanotube array was located. Finally, a graphene-based top electrode on a polydimethylsiloxane (PDMS) structure was placed on the PMMA/Si membrane. How to cite this article : Lee, J. M. et al. Strong interactive growth behaviours in solution-phase synthesis of three-dimensional metal oxide nanostructures. Nat. Commun. 6:6325 doi: 10.1038/ncomms7325 (2015).